Control of single-ligand chemistry on thiolated Au25nanoclusters 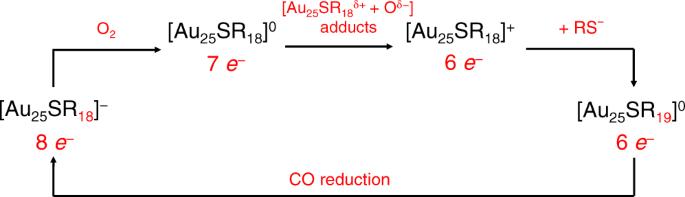Fig. 1: Schematic illustration of reaction process. Schematic illustration of the addition/elimination reaction cycle between [Au25SR18]−and [Au25SR19]0. Diverse methods have been developed to tailor the number of metal atoms in metal nanoclusters, but control of surface ligand number at a given cluster size is rare. Here we demonstrate that reversible addition and elimination of a single surface thiolate ligand (-SR) on gold nanoclusters can be realized, opening the door to precision ligand engineering on atomically precise nanoclusters. We find that oxidative etching of [Au 25 SR 18 ] − nanoclusters adds an excess thiolate ligand and generates a new species, [Au 25 SR 19 ] 0 . The addition reaction can be reversed by CO reduction of [Au 25 SR 19 ] 0 , leading back to [Au 25 SR 18 ] − and eliminating precisely one surface ligand. Intriguingly, we show that the ligand shell of Au 25 nanoclusters becomes more fragile and rigid after ligand addition. This reversible addition/elimination reaction of a single surface ligand on gold nanoclusters shows potential to precisely control the number of surface ligands and to explore new ligand space at each nuclearity. Metal nanoclusters have received tremendous research interests in the past two decades due to their atomically-precise structures, intriguing physicochemical properties, and wide potential applications [1] , [2] , [3] , [4] , [5] . Because of the atomically-precise nature of metal nanoclusters, delicate control of cluster size in synthesis has long been the crucial prerequisite in research [1] , [2] , [3] , [4] , [5] , [6] . Taking thiolate-protected Au nanoclusters as an example, the most traditional and widely-used method is the chemical reduction of Au(I)-thiolate precursors followed by a size-focusing process [7] , [8] . It has been reported that, in the size-focusing process, oxygen (O 2 )-generated thiol radicals can induce the selective etching of metastable intermediates by drawing out Au atoms from the metallic core (i.e., top-down process) [9] . As a result, the polydisperse species will transform to thermodynamically stable monodisperse final products. Thiolate-protected metal nanoclusters are often referred to as [M n SR m ] q (SR denotes thiolate ligands), where n , m , q represent numbers of metal atoms, thiolate ligands and net charge, respectively. The size-focusing will change the n value and result in some thermodynamically stable magic sizes, such as [Au 25 SR 18 ] − . The high stability of [Au 25 SR 18 ] − can be explained by the valence electron counts ( N* = n – m – q ) of 8, which fulfills the shell closing phenomenon [10] . As a result, [Au 25 SR 18 ] − is one of the typical species survived in the size-focusing or ligand-induced etching process [11] , [12] . Its oxidation will simply change the q value from −1 to 0 or +1 and introduce slight distortion into its structure, without changing the total molecular formula [13] , [14] , [15] . Tailoring of surface ligands is equally important considering the total synthesis of metal nanoclusters [6] . The surface ligands will greatly influence the cluster size, as well as physicochemical properties, self-assembly behavior, stability and so on [16] , [17] , [18] , [19] , [20] , [21] , [22] , [23] , [24] , [25] , [26] , [27] . Ligand exchange reaction is the main technique used to tailor the surface ligands of thiolate-protected metal nanoclusters [28] . One possible result of a ligand exchange reaction is partial or total substitution of surface ligands without altering the total formula of the parent cluster [29] , [30] . The other one is the complete change of cluster size, the so-called ligand-exchange-induced size/structure transformation process, which has been applied to discover new cluster species [16] , [31] . However, all the above methodologies have not addressed an important challenge to precisely control the number of surface ligands ( m value) by adding/removing a single ligand at a time for a given number of metal atoms ( n value). To meet the challenge, here we successfully realized the addition and elimination of a surface ligand in thiolate-protected gold nanoclusters based on [Au 25 SR 18 ] − , the flagship cluster of the [M n SR m ] q family. We demonstrated the reversible conversion between water-soluble [Au 25 SR 18 ] − and [Au 25 SR 19 ] 0 nanoclusters with identical thiolate ligand through an oxidative etching/reduction cycle (Fig. 1 ). Detailed evidence from electrospray ionization mass spectrometry (ESI-MS) indicated a continuous oxidation process of the as-prepared [Au 25 SR 18 ] − ( N* = 8) to [Au 25 SR 18 ] 0 ( N* = 7), and then to [Au 25 SR 18 ] + ( N* = 6). [Au 25 SR 18 ] + nanoclusters then reacted with an excess thiolate ligand to form a new isoelectric species, [Au 25 SR 19 ] 0 ( N* = 6), realizing the addition of one thiolate ligand to the original nanocluster. The reverse process can be realized by carbon monoxide (CO)-reduction reaction to eliminate one thiolate ligand in [Au 25 SR 19 ] 0 and regenerate [Au 25 SR 18 ] − . Fig. 1: Schematic illustration of reaction process. Schematic illustration of the addition/elimination reaction cycle between [Au 25 SR 18 ] − and [Au 25 SR 19 ] 0 . Full size image Synthesis of Au nanoclusters [Au 25 (MHA) 18 ] − (MHA = 6-mercaptohexanoic acid) was selected as the model cluster in the oxidative etching exploration. The as-prepared sample clearly shows characteristic absorption peaks of [Au 25 SR 18 ] – (Fig. 2a , 400, 440, 543, 675, and 800 nm) [32] . Electrospray ionization mass spectrometry (ESI-MS) also indicates the successful synthesis of [Au 25 (MHA) 18 ] − species (Fig. 2c ). Note that purification was needed before ESI-MS tests, during which the partial oxidation of [Au 25 (MHA) 18 ] − already took place. As a result, the species captured in ESI-MS were from a mixture of [Au 25 (MHA) 18 ] − and [Au 25 (MHA) 18 ] 0 . Fig. 2: Characterization of the Au 25 species. UV-Vis absorption spectra of as-prepared ( a ) [Au 25 MHA 18 ] – and ( b ) [Au 25 MHA 19 ] 0 . Insets show the digital images of the solution of corresponding species. Red arrows indicate the positions of characteristic absorption peaks. ESI-MS spectra of ( c ) [Au 25 MHA 18 ] – and ( d ) [Au 25 MHA 19 ] 0 . Both experimental and simulated spectra are shown. Dash lines in c are guidelines to judge the relative intensity of corresponding isotopic peaks. The discrepancy between the experimental and simulated result indicate the co-existence of [Au 25 MHA 18 ] – and [Au 25 MHA 18 ] 0 . Full size image Oxidative etching exploration and product identification The as-prepared [Au 25 (MHA) 18 ] − nanoclusters were then dialyzed (with a dialysis membrane of molecular weight cut-off of 5000 Da) and the pH was lowered to 9.0 ± 0.2 to accelerate the oxidation (see Supplementary Fig. 1 ). The characteristic absorption peaks of [Au 25 MHA 18 ] – disappeared completely within 24 h. Polyacrylamide gel electrophoresis (PAGE) was applied to analyze and purify the final product (Supplementary Fig. 2 ). The main product was separated for further characterization. UV-Vis absorption spectrum shows significantly blue-shifted absorption band edge compared to [Au 25 MHA 18 ] – and characteristic absorption peaks at 440, 545, and 585 nm (Fig. 2b ), indicating the formation of a new species. ESI-MS was then applied to determine its molecular formula (Fig. 2d ). The isotope pattern only matched well with [Au 25 MHA 19 ] 0 , a species with the same nuclearity but different ligand number. Thus, it seems possible to precisely adding one thiolate ligand into [Au 25 MHA 18 ] – . Mechanism of the ligand addition reaction To further verify this addition reaction and examine its mechanism, we simplified the whole reaction system by removing the excess ligands, Au(I)-complexes and inorganic ions remained in the solution using PAGE separation. These species may cause the side reactions and the formation of by-products, and a typical dialysis may not be able to completely remove them. The absorption spectrum of the purified [Au 25 MHA 18 ] species was shown in Fig. 3a . Fig. 3: Monitoring of reaction intermediates. a UV-Vis absorption and b ESI-MS spectra of [Au 25 MHA 18 ] species after PAGE purification and long-time exposure in air. Detailed analysis of the enlarged parts in red and blue square is shown in c and d , respectively. Both experimental and simulated isotopic patterns of labeled species are included. Full size image ESI-MS was then applied to monitor the variation of [Au 25 MHA 18 ] species after the long-time exposure in air. The overall spectrum indicates the high purity of [Au 25 MHA 18 ] species (Fig. 3b ). However, in a detailed analysis of isotopic patterns (Fig. 3c ), we found that the majority of [Au 25 MHA 18 ] species have been oxidized from [Au 25 MHA 18 ] – ( N* = 8) to [Au 25 MHA 18 ] 0 ( N* = 7). Furthermore, we noticed an excess small peak that can only be assigned to [Au 25 MHA 18 ] + ( N* = 6), product originated from the further oxidation of [Au 25 MHA 18 ] species. Actually, it is the first time that the water-soluble [Au 25 SR 18 ] was found to be oxidized to the valence state of +1 [13] . As no external oxidant was added to the solution to induce the reaction, the only oxidation resource in this reaction should be O 2 in the air. The signals shown in Fig. 3d further support this conjecture. We clearly observed the signals which could be assigned to [Au 25 MHA 18 δ+ + O δ− ] adducts. This assignment was supported by the fact that these signals become stronger after introducing excess oxidation reagent such as H 2 O 2 (Supplementary Fig. 3 ). The [Au 25 MHA 18 δ+ + O δ− ] adducts should be the intermediate in the reaction between molecular O 2 and [Au 25 MHA 18 ] nanoclusters to generate [Au 25 MHA 18 ] + . Further prolonging the oxidation reaction time will not increase the abundance of [Au 25 MHA 18 ] + (Supplementary Fig. 4a ), indicating an equilibrium between [Au 25 MHA 18 ] 0 and [Au 25 MHA 18 ] + species. However, introducing reducing reagent such as CO and oxidation reagent such as H 2 O 2 will suppress and increase the signals corresponding to [Au 25 MHA 18 ] + , respectively, further confirming our assignments (Supplementary Fig. 4b and 4c ). Since [Au 25 MHA 18 ] + and final product [Au 25 MHA 19 ] 0 have the same N* value of 6, oxidation is not needed in subsequent transformation process. At this stage, [Au 25 MHA 18 ] + reacting with one free thiol ligand will drive the isoelectric reaction to the final product [Au 25 MHA 19 ] 0 . Reversible conversion process We thus introduced excess thiol ligands into the solution and monitor the transformation process by UV-vis absorption spectroscopy and real-time ESI-MS. We observed two isosbestic points in the UV-vis absorption spectra at 536 and 627 nm (Fig. 4a ), which indicates a quasi-one-to-one transformation process (Supplementary Note 1). The ESI-MS spectra (Fig. 4b ) also showed a gradual consuming of [Au 25 MHA 18 ] species and generating of [Au 25 MHA 19 ] 0 without other observable intermediates. The final product was shown to be pure [Au 25 MHA 19 ] 0 nanoclusters (Supplementary Fig. 5 ). Thus, we have successfully demonstrated that one thiolate ligand can be precisely added to one [Au 25 MHA 18 ] − to form a [Au 25 MHA 19 ] 0 . Fig. 4: Interconversion process. a Time-course UV-Vis absorption spectra and b ESI-MS spectra in the transformation from [Au 25 MHA 18 ] species to [Au 25 MHA 19 ] 0 after introducing excess thiol ligands. c and d show the oxidative etching/reduction cycles between [Au 25 MHA 18 ] – and [Au 25 MHA 19 ] 0 by UV-vis absorption spectra and normalized absorbance at 675 nm in the reversible transformation process, respectively. Full size image As many chemical reactions are reversible in nature, we then investigated the possibilities to precisely eliminate one ligand from [Au 25 MHA 19 ] 0 to [Au 25 MHA 18 ] − . We were able to realize this transformation by introducing a reducing agent, CO, to [Au 25 MHA 19 ] 0 solution. Pure [Au 25 MHA 18 ] – was formed as indicated by UV-Vis absorption and ESI-MS spectra (Supplementary Fig. 6 ). Furthermore, the oxidative etching of [Au 25 MHA 18 ] – and reduction of [Au 25 MHA 19 ] 0 can be reversibly realized (Fig. 4c, d ) by simply tailoring the pH of the solution and atmosphere (pH ~9, air for oxidative etching and pH ~12, CO for reduction). Change of ligand number on the same nuclearity will inevitably influence the structure of ligand shell and thus the properties of whole nanocluster. We try to gain further insights into differences of the ligand shell after addition/elimination of one excess thiolate ligand using tandem mass spectrometry and nuclear magnetic resonance (NMR) analysis. Tandem mass spectrometry has been widely applied in structural analysis of molecular-like clusters and shows sensitivity in analyzing the surface motifs [33] , [34] . As shown in Fig. 5a, b , the onset energy of fragmentation decreased dramatically from 20 eV of [Au 25 MHA 18 ] species (dominant species: [Au 25 MHA 18 ] 0 ) to 5 eV of [Au 25 MHA 19 ] 0 , indicating a more fragile nature of the surface structure after addition of one excess thiolate ligand. However, these two species showed a similar fragment pattern that the major fragmentation routes are the same by dissociation of one Au 4 SR 4 unit stepwise in 1st and 2nd generation fragmentation. In addition, a less prominent 1 st generation fragment of [Au 25 MHA 19 ] 0 by dissociation of one Au 5 SR 5 unit has been detected, which should be the result of lengthened motif after ligand addition. Fig. 5: Tandem mass testing of the Au 25 species. Tandem mass spectra and corresponding fragmentation patterns of ( a ) [Au 25 MHA 18 ] and ( b ) [Au 25 MHA 19 ] 0 . ( m , n ) denotes species with molecular formula of Au m SR n . Different routes are divided into major, minor, and trace categories based on the abundance in tandem mass spectra. See Supplementary Fig. 7 and 8 for detailed assignments of fragment species. Full size image 1 H-NMR signals of surface protecting ligands also provide substantial information of ligand shell in metal nanoclusters [35] , [36] , [37] . As shown in Fig. 6 , the signals of protons in MHA surface ligands can be well assigned into two sets in [Au 25 MHA 18 ] − (see Supplementary Fig. 9 for assignments of the two kinds of surface ligands). Note that NaBH 4 was introduced to reduce the [Au 25 MHA 18 ] species to −1 state to get a more analyzable spectrum. In the spectrum of [Au 25 MHA 19 ] 0 , the most obvious differences of the signals were the largely broadened and smoothened peaks. The broadened and featureless signals were the direct result of limited motion of surface ligands [38] , indicating a more rigidified ligand shell after addition of one excess thiolate ligand. Note that the peak broadening can also be the result of a distribution of isotropic chemical shift (typically observed in larger metal nanoparticles) [39] , a paramagnetic core (observed in metal nanoclusters with odd N * together with huge down-shift of NMR signals) and electron transfer between different oxidation states of metal nanoclusters [40] , which are not expected to exist in [Au 25 MHA 19 ] 0 . Fig. 6: 1 H-NMR testing of the ligand shell. 1 H-NMR spectra of MHA ligand, [Au 25 MHA 18 ] − , and [Au 25 MHA 19 ] 0 . Sharp peaks around chemical shift of 3.30 and 2.40 ppm are from impurities introduced in PAGE and ultrafiltration process which are hard to be removed and assigned. 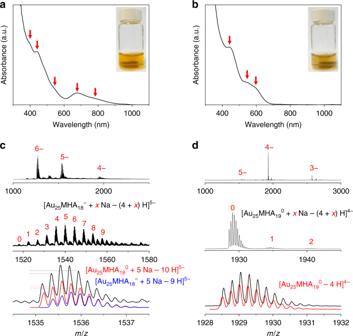Fig. 2: Characterization of the Au25species. UV-Vis absorption spectra of as-prepared (a) [Au25MHA18]–and (b) [Au25MHA19]0. Insets show the digital images of the solution of corresponding species. Red arrows indicate the positions of characteristic absorption peaks. ESI-MS spectra of (c) [Au25MHA18]–and (d) [Au25MHA19]0. Both experimental and simulated spectra are shown. Dash lines incare guidelines to judge the relative intensity of corresponding isotopic peaks. The discrepancy between the experimental and simulated result indicate the co-existence of [Au25MHA18]–and [Au25MHA18]0. Full size image Summing up the experimental evidence above, we think that the single-ligand chemistry and the interconversion of [Au 25 SR 18 ] – and [Au 25 SR 19 ] 0 can be described by the following two reactions: 
    [ Au_25SR_18]^ - + 1/2   O_2 + HSR→[ Au_25SR_19]^0  + OH^ -
 (1) 
    [ Au_25SR_19]^0 + CO + 2OH^ - →[ Au_25SR_18]^ - + HCO_3^ -  + HSR. (2) Energetics for the two reactions can be computed by density functional theory (DFT) and help understand the thermodynamic driving force of the two reactions. To this end, a structural model for [Au 25 SR 19 ] 0 would be needed. Given the similar patterns in tandem mass spectra of [Au 25 SR 18 ] and [Au 25 SR 19 ] 0 , we hypothesize that they have a similar ligand shell composition. Indeed, we found that the structural model with a defective icosahedral core and lengthened Au 3 SR 4 motif is more stable than many other isomers that we tested (Supplementary Fig. 10 ; see Supplementary information for computational details). We therefore used this model as our putative structure for [Au 25 SR 19 ] 0 when computing the reaction energetics. (Here we note that a total structure prediction for [Au 25 SR 19 ] 0 is still computationally demanding and beyond the scope of this work). The computed ΔE at the B3LYP/TZVP level with an implicit solvation model is −0.11 eV for reaction (1) and −4.57 eV for reaction (2), in qualitative agreement with our experimental observation. In other words, when pH is lowered, a single thiol (HSR) ligand can be oxidatively added to [Au 25 SR 18 ] – under O 2 with a favorable energy gain, while [Au 25 SR 19 ] 0 can be reduced back to [Au 25 SR 18 ] – by CO at higher pH at more favorable energetics. Besides the favorable energetic of the transformation from [Au 25 SR 18 ] – to [Au 25 SR 19 ] 0 under the oxidative environment in the presence of free thiol ligands, [Au 25 MHA 19 ] 0 also shows higher resistance to oxidative etching than [Au 25 MHA 18 ] – (Supplementary Fig. 11 ). The enhanced stability of [Au 25 MHA 19 ] 0 under the oxidative environment is probably due to the lengthened motifs and rigidified ligand shell, which will provide better protection to the Au(0) core and prevent the access of oxidative species (e.g., O 2 and thiol radicals). Thus, we were able to obtain the pure product of [Au 25 MHA 19 ] 0 by the as-speculated oxidative etching reaction. In conclusion, we successfully demonstrated a reaction cycle composed of precise addition and elimination of one thiolate surface ligand on gold nanoclusters. The addition of one thiolate ligand into the original [Au 25 MHA 18 ] – nanoclusters was realized by an oxidative etching reaction. In this process, [Au 25 MHA 18 ] – was first oxidized by O 2 stepwise from −1 state to 0 and +1 state. The [Au 25 MHA 18 ] + then reacted with one free thiol ligand to generate [Au 25 MHA 19 ] 0 . Tandem mass spectrometry and 1 H-NMR indicated that addition of one excess ligand resulted in a ligand shell with similar composition, but more fragile and rigid. We further realized the reverse process by CO-reduction, eliminating one thiolate surface ligand and regenerating [Au 25 MHA 18 ] – nanoclusters. Computed reaction energetics from DFT confirms the driving force of the ligand chemistry and the interconversion of [Au 25 MHA 18 ] – and [Au 25 MHA 19 ] 0 . The key point of such manipulation should be using a stoichiometric amount of ligands in the oxidative etching reaction, which creates a mild reaction condition to possibly stabilize the metastable products. This method provides more opportunities in discovery of ‘hidden’ species at a given nanocluster size (or metal atom number) with precisely controlled surface ligand number and surface rigidity, and generating new physical and chemical properties, such as photoluminescence and catalysis. Materials 6-mercaptohexanoic acid (MHA), were purchased from Sigma-Aldrich. Hydrogen tetrachloroaurate(III) hydrate (HAuCl 4 ·3H 2 O) was purchased from Alfa Aesar. Sodium hydroxide (NaOH) was purchased from Sigma-Aldrich. Carbon monoxide (CO, 99.9%) was obtained from Singapore Oxygen Air Liquide Pte Ltd (SOXAL). All chemicals were used without further purification. Ultrapure water (18.2 MΩ cm) was used in all the experiments. All glassware was washed with aqua regia before use. Synthesis of [Au 25 (MHA) 18 ] − nanoclusters [Au 25 (MHA) 18 ] − nanoclusters were synthesized through a CO-reduction method. In a typical synthesis, 4 mL of aqueous solution of 5 mM MHA and 0.2 mL of aqueous solution of 50 mM HAuCl 4 were added into 5.8 mL of ultrapure water. After 5 min, the pH of the solution was brought up to 12.0 by dropwise adding aqueous solution of 1 M NaOH. After 30 min, CO was bubbled into the solution for 2 min. The reaction vessel was then kept airtight and the reaction was allowed to proceed for 24 h under gentle stirring (500 rpm) at room temperature. The raw product was either purified by ultrafiltration (membrane of molecular weight cut-off = 5000 Da) before testing electrospray ionization mass spectrometry (ESI-MS), or purified by dialysis (membrane of molecular weight cut-off = 5000 Da) before further oxidation reaction. Native polyacrylamide gel electrophoresis (PAGE) separation of the Au nanoclusters In the native PAGE experiments, Bio-Rad Mini-PROTEAN® Tetra Cell or PROTEAN® II xi Cell system was used. Stacking and resolving gels were prepared by 4 and 30 wt% acrylamide monomers (1:19), respectively. The Au nanocluster solutions were first concentrated by ultrafiltration and then mixed with glycerol to prepare the sample solutions (~10 mM based on Au atoms, 50 vol% glycerol). 2 mL of sample solution were loaded into the well. The PAGE was conducted with constant voltage of 180 V for 24 h at 4 °C. The bands were cut, crushed, and incubated in ultrapure water to obtain solutions of pure Au nanoclusters for further use. The cluster concentration was determined by inductively coupled plasma mass spectrometry (ICP-MS) measurements. Conversion from purified [Au 25 (MHA) 18 ] species to [Au 25 (MHA) 19 ] 0 Purified [Au 25 (MHA) 18 ] species from PAGE were used. In a typical reaction, 1 equivalent excess MHA (40 μM) was introduced into the solution of [Au 25 (MHA) 18 ] (~ 1 mM of [Au]). The solution pH was adjusted to 9.0 ± 0.2. Time-course absorption spectra and ESI-MS spectra were then recorded. Note that the reaction was conducted without stirring in time-course monitoring, and will be accelerated if stirring was applied (completed within 24 h). Conversion from [Au 25 (MHA) 19 ] 0 to [Au 25 (MHA) 18 ] − by CO reduction The solution pH was brought up to 12.0 by an aqueous solution of 1 M NaOH. CO was bubbled into the solution for 2 min. The reaction was proceeded for 12 h airtight. The sample needs to be purified by ultrafiltration before ESI-MS test. Characterizations Solution pH was recorded by Mettler-Toledo FE 20 pH-meter. UV-vis absorption spectra were recorded by Shimadzu UV-1800 spectrometer. ESI-MS spectra were captured by a Bruker microTOF-Q system in negative ion mode. 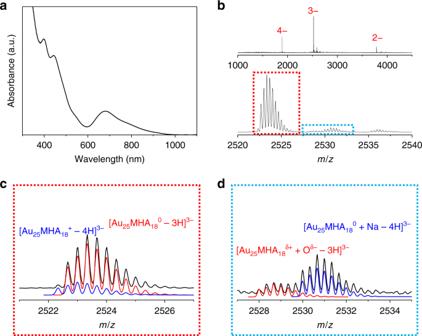Fig. 3: Monitoring of reaction intermediates. aUV-Vis absorption andbESI-MS spectra of [Au25MHA18] species after PAGE purification and long-time exposure in air. Detailed analysis of the enlarged parts in red and blue square is shown incandd, respectively. Both experimental and simulated isotopic patterns of labeled species are included. 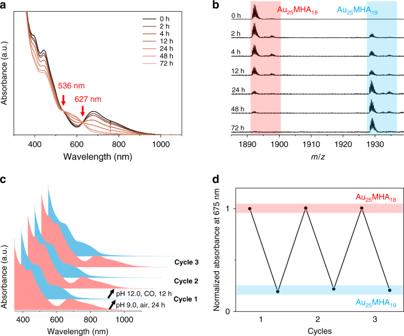Fig. 4: Interconversion process. aTime-course UV-Vis absorption spectra andbESI-MS spectra in the transformation from [Au25MHA18] species to [Au25MHA19]0after introducing excess thiol ligands.canddshow the oxidative etching/reduction cycles between [Au25MHA18]–and [Au25MHA19]0by UV-vis absorption spectra and normalized absorbance at 675 nm in the reversible transformation process, respectively. ESI-MS testing parameters: source temperature 120 °C, dry gas flow rate 8 L per min, nebulizer pressure 3 bar, capillary voltage 3.5 kV, and sample injection rate 3 μL per min. 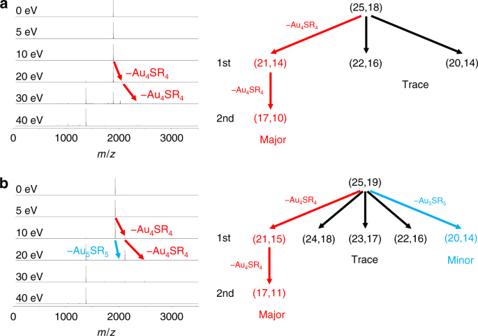Fig. 5: Tandem mass testing of the Au25species. Tandem mass spectra and corresponding fragmentation patterns of (a) [Au25MHA18] and (b) [Au25MHA19]0. (m,n) denotes species with molecular formula of AumSRn. Different routes are divided into major, minor, and trace categories based on the abundance in tandem mass spectra. See Supplementary Fig. 7 and 8 for detailed assignments of fragment species. 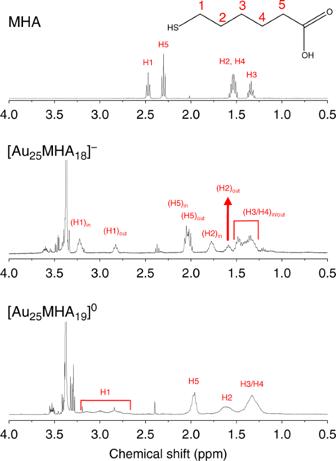Fig. 6:1H-NMR testing of the ligand shell. 1H-NMR spectra of MHA ligand, [Au25MHA18]−, and [Au25MHA19]0. Sharp peaks around chemical shift of 3.30 and 2.40 ppm are from impurities introduced in PAGE and ultrafiltration process which are hard to be removed and assigned. In ESI-MS test, the solution was directly injected without further purification unless specified. 1 H-NMR spectra were recorded on Bruker 400 MHz system using D 2 O as solvent. Purified samples were obtained from PAGE separation and further ultrafiltration process.